Orbitofrontal lesions eliminate signalling of biological significance in cue-responsive ventral striatal neurons The ventral striatum has long been proposed as an integrator of biologically significant associative information to drive actions. Although inputs from the amygdala and hippocampus have been much studied, the role of prominent inputs from orbitofrontal cortex (OFC) are less well understood. Here, we recorded single-unit activity from ventral striatum core in rats with sham or ipsilateral neurotoxic lesions of lateral OFC, as they performed an odour-guided spatial choice task. Consistent with prior reports, we found that spiking activity recorded in sham rats during cue sampling was related to both reward magnitude and reward identity, with higher firing rates observed for cues that predicted more reward. Lesioned rats also showed differential activity to the cues, but this activity was unbiased towards larger rewards. These data support a role for OFC in shaping activity in the ventral striatum to represent the biological significance of associative information in the environment. The ventral striatum (VS) has long been proposed as an area critical to integrating affective information to drive actions [1] , [2] , [3] , [4] , [5] . This role is evident in numerous single-unit recording studies [6] , [7] , [8] , [9] , [10] , [11] , [12] , [13] , [14] , which typically find that activity in this area is driven by some combination of the associative significance or value of cues and the required responses, and in the many well-controlled behaviours that depend on this region, such as Pavlovian-to-instrumental transfer (PIT) [15] , [16] , [17] , [18] . While the role of input from afferent regions such as the amygdala and hippocampus has been explored [4] , [5] , [19] , [20] , [21] , [22] , [23] , [24] , relatively little attention has been given to the prominent input this area receives from the orbitofrontal cortex (OFC). OFC sends extensive input to the VS [25] , [26] , [27] , [28] , [29] , and the OFC serves a role in behaviour and decision-making that is somewhat similar though not identical to that of the VS. For example, like VS, the OFC is thought to signal biologically significant associative information [30] , [31] , [32] . However, while the VS is necessary for both general and specific forms of PIT [15] , [16] , [17] , [18] , the OFC has thus far been implicated in only specific, but not general, PIT [33] . Likewise, VS is necessary for unblocking based on either value or identity information, whereas the OFC is only necessary for identity-based unblocking [34] . These partial dissociations raise interesting questions regarding which representations in VS depend on OFC and which might be OFC-independent. To investigate this question, we recorded single-unit activity from VS core in rats with ipsilateral sham or neurotoxic lesions of the lateral OFC. We chose VS core because this region appears to receive the heaviest direct input from lateral OFC in rats [25] , [26] , [27] , [28] , [29] . Recordings were made as rats performed a simple odour-guided choice task, in which odours served as cues for the spatial location of the reward (left or right well). During each recording session, the identity and number of rewards in each well was manipulated across blocks of trials. We found that neurons in sham rats showed differential activity to the cues that reflected the number of rewards and the direction of the required response. Much of this activity seemed value related, inasmuch as higher firing was typically observed to the larger reward. In addition, we also found ample representation of value combined with reward identity. Lesioned rats also showed differential activity to the cues, but this activity was largely devoid of a bias towards representing larger or more valuable rewards. These data support a role for the OFC in biasing activity in the VS core to represent the biological significance of associative information in the environment. This role is consistent with anatomical and behavioural evidence and provides novel insight regarding how orbital regions may influence downstream processing. Neurons were recorded during performance of an odour-guided choice task (illustrated in Fig. 1a ). In this task, odour cues signalled the rat to respond left or right to receive small (one drop of ∼ 0.05 ml) or large (three drops) amounts of two equally preferred chocolate- or vanilla-flavoured milk solutions (see Fig. 1b ). Response-reward contingencies were stable across blocks of ∼ 60 trials, but switched unpredictably between blocks. Contingencies were arranged so that (1) rewards in the two directions always differed in both number and flavour (for example, large chocolate versus small vanilla or large vanilla versus small chocolate) and (2) number and flavour switches alternated according to the sequence number-flavour-number-flavour across the five blocks of every session. After initial shaping to proficiency on the task (see Methods), rats received unilateral sham ( n =4) or neurotoxic lesions ( n =5; Fig. 1c ) of the lateral OFC, and electrode arrays were implanted in ipsilateral VS core. After recovery, rats were retrained and then recording begun. 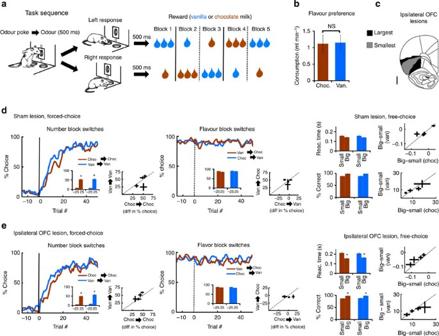Figure 1: Task and behaviour. (a) After initiating a trial with a nose poke and receiving an instructional odour, rats responded at one of two fluid wells for 1 or 3 drops of chocolate (choc) or vanilla (van) milk, delivered 500 ms after the well-poke. Two odours indicated forced choices, left or right; a third odour indicated free choice. Reward contingencies were stable across blocks of∼60 trials, but switched in number of drops (dashed lines) or flavour (dotted lines) in four unsignalled transitions. Rewards in the two directions always differed in both number and flavour (only one of four possible block sequences is shown). (b) Chocolate and vanilla milk solutions were equally preferred in a 10-min consumption test conducted previously in a separate group of rats (mean±s.e.;n=6;t10=0.1,P=0.93). (c) Shown is the extent of unilateral neurotoxic lesions of orbitofrontal cortex (OFC) made in one group. (d) Control rats (sham lesions) were sensitive to the number of drops but not the flavour of reward (n=83 sessions). Number switches (left panel,d) had a large effect on choice rates independent of flavour. Flavour switches (middle panel,d) had no effect on choice rates for big vanilla to big chocolate or big chocolate to big vanilla switches. Line figures show average trial-by-trial choice rates; inset bar graphs compare average choice rates±s.e. in the 25 trials before block switches versus the 25 trials after. In the rightmost panels ofd, reaction (reac.) time (odour offset to port exit; top panel) and accuracy (bottom panel) on forced-choice trials reflected number but not flavour. Scatter plots in each panel show rat-by-rat difference (diff) scores; the length of lines in each dimension represents the s.e. No rat showed a significant effect of flavour on any measure. (e) Rats with unilateral OFC lesions were also sensitive to number but not flavour (n=67 sessions). Their behaviour was not significantly different from shams, except that they had slower reaction times across all conditions and showed a greater effect of number on reaction time. Panels inefollow the same conventions as those ind. No individual rat showed a significant effect of flavour on any measure. Figure 1: Task and behaviour. ( a ) After initiating a trial with a nose poke and receiving an instructional odour, rats responded at one of two fluid wells for 1 or 3 drops of chocolate (choc) or vanilla (van) milk, delivered 500 ms after the well-poke. Two odours indicated forced choices, left or right; a third odour indicated free choice. Reward contingencies were stable across blocks of ∼ 60 trials, but switched in number of drops (dashed lines) or flavour (dotted lines) in four unsignalled transitions. Rewards in the two directions always differed in both number and flavour (only one of four possible block sequences is shown). ( b ) Chocolate and vanilla milk solutions were equally preferred in a 10-min consumption test conducted previously in a separate group of rats (mean±s.e. ; n =6; t 10 =0.1, P =0.93). ( c ) Shown is the extent of unilateral neurotoxic lesions of orbitofrontal cortex (OFC) made in one group. ( d ) Control rats (sham lesions) were sensitive to the number of drops but not the flavour of reward ( n =83 sessions). Number switches (left panel, d ) had a large effect on choice rates independent of flavour. Flavour switches (middle panel, d ) had no effect on choice rates for big vanilla to big chocolate or big chocolate to big vanilla switches. Line figures show average trial-by-trial choice rates; inset bar graphs compare average choice rates±s.e. in the 25 trials before block switches versus the 25 trials after. In the rightmost panels of d , reaction (reac.) time (odour offset to port exit; top panel) and accuracy (bottom panel) on forced-choice trials reflected number but not flavour. Scatter plots in each panel show rat-by-rat difference (diff) scores; the length of lines in each dimension represents the s.e. No rat showed a significant effect of flavour on any measure. ( e ) Rats with unilateral OFC lesions were also sensitive to number but not flavour ( n =67 sessions). Their behaviour was not significantly different from shams, except that they had slower reaction times across all conditions and showed a greater effect of number on reaction time. Panels in e follow the same conventions as those in d . No individual rat showed a significant effect of flavour on any measure. Full size image During recording, rats in both groups attended to differences in reward number but not flavour. Thus, number switches resulted in a rapid and sustained change in choice rate on free-choice trials ( Fig. 1d,e , left panels), and the rate of switching was independent of flavour and lesion status (see Supplementary Table 1 for statistics). In addition, reaction time was faster and performance was more accurate on forced-choice trials when a large reward was at stake ( Fig. 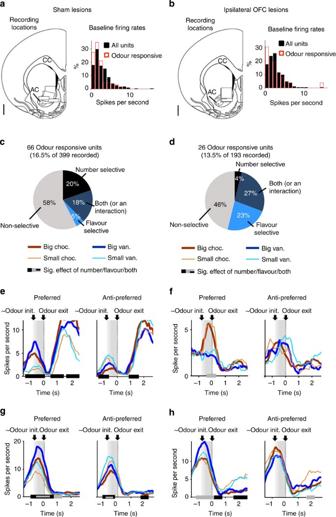Figure 2: Single-unit recordings of odour-responsive units. (a,b) Shown are recording locations and baseline firing rate distributions in the sham (a) and OFC-lesioned groups (b). The width of each box (1 mm) represents the approximate spread of recording wires, and the height represents the estimated range through which the bundle was driven during recording sessions. Each box represents one rat. Scale bar, 1 mm. AC, anterior commissure; CC, corpus callosum. Baseline firing rates were not significantly different in the two groups, for either the whole population (t590=−0.15,P=0.88) or in the odour-responsive population, (t90=−1.5,P=0.13). (c,d) Pie charts represent all odour-responsive units (defined as those with a significant (sig.) increase over baseline during the odour epoch). Coloured sections represent units with significant effects of number (black), flavour (blue) or both (cross-hatched), based on an analysis of variance (ANOVA) on firing rate in that unit’s preferred direction during the odour epoch. There was no significant difference in the proportion of odour-responsive units in the two groups (by chi-square,P=0.25). However, with OFC lesions, units were significantly more likely to be flavour-selective and significantly less likely to be number-selective with no effect of flavour (chi-square on distribution of units across these categories,P<0.0001). Indeed, by chi-square, in the sham group, the number of purely flavour-selective neurons (with no effect of number) was not significantly different from chance (P=0.74), while the number of purely number-selective neurons was significantly greater than chance (P<0.00001); in the lesion group, the opposite was true (purely flavour-selective,P<0.00001; purely number-selective,P=0.90). (e–h) Single-unit examples from the sham (e,g) and lesion groups (f,h). Black and grey bars indicate bins with a significant effect of number or flavour, respectively, by ANOVA on a sliding average of five bins. Significant effects were found mostly on the preferred side (left side of each panel). Units in the sham group tended to prefer the odours predicting large outcomes, in some cases with no effect of flavour (e) and in other cases with an additional effect of flavour (g). Units in the lesion group were more likely to be flavour-selective without a strong effect of number. choc., chocolate; init., initiation; van., vanilla. 1d,e , right panels; see Supplementary Table 2 for statistics). Again, these effects were independent of reward flavour and did not differ on the basis of lesion status, although there was a general increase in reaction time in lesioned rats. Importantly, changes in behaviour driven by reward number were similar for the two milk flavours for each individual rat analysed separately, and switches between flavours had no effect on choice rate for each individual rat analysed separately (see scatter plots in Fig. 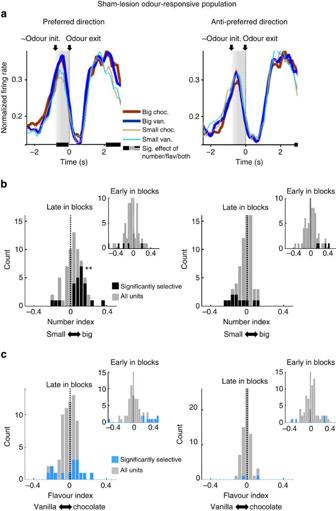Figure 3: Outcome selectivity in ventral striatum of sham-lesioned rats. (a) Shown are population averages of normalized firing rate across the time of the trial, aligned to the end of the odour period, for all odour-responsive units (n=66). Activity is averaged by preferred (left panel) and anti-preferred (right panel) directions, and by the specific reward available at the end of the trial (in different colours). Preferred direction was defined for each unit by the direction with the highest average activity during the epoch from odour initiation (init.) to port withdrawal (in grey shading). Only correct forced-choice trials in the latter part of the block (after the first 20 correct trials) are included in the averages. Black bars indicate bins with a significant (sig.) effect of number of drops of reward, by ANOVA on a sliding average of five bins across neurons. There were no bins with a significant effect of reward flavour (flav). (b) Shown are number-selectivity indices during the odour epoch for each neuron in the population, separately for the preferred (left panels) and anti-preferred (right panels) directions. Insets show indices early in blocks immediately following number shifts. Number-selectivity index was defined as the difference in normalized firing rate between conditions with the large reward and those with the small reward. Dark-coded units are those in which this difference was significant across trials. **P<0.01, both the indices of the population and the proportion of significant neurons were significantly shifted to the right. (c) Shown are flavour-selectivity indices with the same conventions as inb., with insets showing the indices in the trials immediately after flavour shifts. Indices were not shifted towards either flavour (except early in the preferred direction), but had a larger magnitude (absolute value) and were more likely to be significant, in the preferred direction compared with the anti-preferred, late in blocks. choc., chocolate; van., vanilla. 1d,e , and Supplementary Table 3 for statistics). Thus performance on both free- and forced-choice trials was sensitive to reward number, reflecting the higher value of a large reward, but insensitive to flavour, reflecting the similar value placed on chocolate and vanilla. These effects were observed in both groups and within each individual rat, and there was no effect of unilateral lesions. Activity integrates response direction and reward number We recorded 592 single units in VS core of sham and lesioned rats; recording locations and baseline firing rats were similar across groups ( Fig. 2a,b ). We were particularly interested in cue-evoked activity; such activity in VS has been frequently reported to encode associative information. For example, in a prior study in which we manipulated both the number and timing of reward, we found that cue-evoked activity was heavily influenced by these two variables [6] . Here, we found very similar effects in sham rats. As in the previous study, we defined the preferred direction for each unit as that for which firing rate during the cue epoch was highest across all conditions, and then tested for effects of the associated reward in that direction. Within the cue-responsive population (66 of 399 total single units recorded in sham rats), almost a quarter of the neurons (13) exhibited a main effect of number with no accompanying effect of flavour, and an approximately equal number (12) exhibited a number-by-flavour interaction or main effects of both number and flavour in their cue-evoked firing ( Fig. 2c ). The response-specific influence of reward number was evident in the evoked activity of individual units, which tended to fire most to the cues that predicted the high magnitude reward in a particular direction ( Fig. 2e,g ). Notably, very few units responded differentially on the basis of flavour alone ( Fig. 2c ). See Table 1 for a full accounting of neuron categorization and statistics. Figure 2: Single-unit recordings of odour-responsive units. ( a , b ) Shown are recording locations and baseline firing rate distributions in the sham ( a ) and OFC-lesioned groups ( b ). The width of each box (1 mm) represents the approximate spread of recording wires, and the height represents the estimated range through which the bundle was driven during recording sessions. Each box represents one rat. Scale bar, 1 mm. AC, anterior commissure; CC, corpus callosum. Baseline firing rates were not significantly different in the two groups, for either the whole population ( t 590 =−0.15, P =0.88) or in the odour-responsive population, ( t 90 =−1.5, P =0.13). ( c , d ) Pie charts represent all odour-responsive units (defined as those with a significant (sig.) increase over baseline during the odour epoch). Coloured sections represent units with significant effects of number (black), flavour (blue) or both (cross-hatched), based on an analysis of variance (ANOVA) on firing rate in that unit’s preferred direction during the odour epoch. There was no significant difference in the proportion of odour-responsive units in the two groups (by chi-square, P =0.25). However, with OFC lesions, units were significantly more likely to be flavour-selective and significantly less likely to be number-selective with no effect of flavour (chi-square on distribution of units across these categories, P <0.0001). Indeed, by chi-square, in the sham group, the number of purely flavour-selective neurons (with no effect of number) was not significantly different from chance ( P =0.74), while the number of purely number-selective neurons was significantly greater than chance ( P <0.00001); in the lesion group, the opposite was true (purely flavour-selective, P <0.00001; purely number-selective, P =0.90). ( e – h ) Single-unit examples from the sham ( e , g ) and lesion groups ( f , h ). Black and grey bars indicate bins with a significant effect of number or flavour, respectively, by ANOVA on a sliding average of five bins. Significant effects were found mostly on the preferred side (left side of each panel). Units in the sham group tended to prefer the odours predicting large outcomes, in some cases with no effect of flavour ( e ) and in other cases with an additional effect of flavour ( g ). Units in the lesion group were more likely to be flavour-selective without a strong effect of number. choc., chocolate; init., initiation; van., vanilla. Full size image Table 1 Number of significantly selective neurons in each condition. Full size table The number-related activity was also evident in the population response of the cue-responsive neurons, which showed higher firing to the larger outcome in the preferred direction, with no overall effect of flavour ( Fig. 3a ). Note that, we also saw, in some neurons, a strong phasic response occurring later in trial, at about the time of the reward, which appears in the population plot. However, unlike number-related activity during the cue, reward-responsive activity was not consistently found across the sham rats in our data set, and thus we did not analyse these responses further (mixed analysis of variance (ANOVA) comparing activity during baseline and reward epoch, with between-subjects factor rat, found only a marginal effect of reward versus baseline, F 1,62 =3.3, P =0.07, and a large interaction between reward versus baseline and rat, F 3,62 =26.5, P <0.000001; across units from some individual rats, activity during the reward epoch was significantly lower than baseline ( n =2), while in only one rat was it higher than baseline). Figure 3: Outcome selectivity in ventral striatum of sham-lesioned rats. ( a ) Shown are population averages of normalized firing rate across the time of the trial, aligned to the end of the odour period, for all odour-responsive units ( n =66). Activity is averaged by preferred (left panel) and anti-preferred (right panel) directions, and by the specific reward available at the end of the trial (in different colours). Preferred direction was defined for each unit by the direction with the highest average activity during the epoch from odour initiation (init.) to port withdrawal (in grey shading). Only correct forced-choice trials in the latter part of the block (after the first 20 correct trials) are included in the averages. Black bars indicate bins with a significant (sig.) effect of number of drops of reward, by ANOVA on a sliding average of five bins across neurons. There were no bins with a significant effect of reward flavour (flav). ( b ) Shown are number-selectivity indices during the odour epoch for each neuron in the population, separately for the preferred (left panels) and anti-preferred (right panels) directions. Insets show indices early in blocks immediately following number shifts. Number-selectivity index was defined as the difference in normalized firing rate between conditions with the large reward and those with the small reward. Dark-coded units are those in which this difference was significant across trials. ** P <0.01, both the indices of the population and the proportion of significant neurons were significantly shifted to the right. ( c ) Shown are flavour-selectivity indices with the same conventions as in b ., with insets showing the indices in the trials immediately after flavour shifts. Indices were not shifted towards either flavour (except early in the preferred direction), but had a larger magnitude (absolute value) and were more likely to be significant, in the preferred direction compared with the anti-preferred, late in blocks. choc., chocolate; van., vanilla. Full size image To quantify number-related activity during the cue, we calculated a number index score comparing firing in each neuron on the basis of reward number, in both the preferred and anti-preferred direction, and both early and late in blocks. We calculated the score both as a simple subtraction index (the difference between mean normalized firing rates in high versus low reward number conditions) and as a t-statistic comparing firing rates across trials in the two conditions. As shown in these figures, activity biased toward the cue predicting the larger magnitude reward was not present early in the trial blocks following a switch in number, but appeared later ( Fig. 3b and Table 2 for full statistics; see Supplementary Fig. 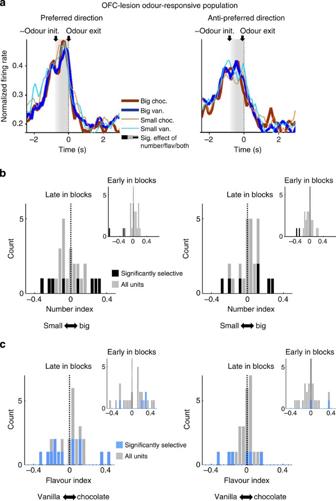Figure 4: Outcome selectivity in ventral striatum of OFC-lesioned rats. (a) Shown are population averages of normalized firing rate across the time of the trial, aligned to the end of the odour period, for all odour-responsive units (n=26). Activity is averaged by preferred (left panel) and anti-preferred (right panel) directions, and by the specific reward available at the end of the trial (in different colours). Preferred direction was defined for each unit by the direction with the highest average activity during the epoch from odour initiation to response initiation (in grey shading). Only correct forced-choice trials in the latter part of the block (after the first 20 correct trials) are included in the averages. There were no bins with significant (sig.) effects of number or flavour (flav), by ANOVA on a sliding average of five bins across neurons. (b) Shown are number-selectivity indices during the odour epoch for each neuron in the population, separately for the preferred (left panels) and anti-preferred (right panels) directions. Insets show indices early in blocks immediately following number shifts. Number-selectivity index was defined as the difference in normalized firing rate between conditions with the large reward and those with the small reward. Dark-coded units are those in which this difference was significant across trials. Unlike in controls, indices were not more likely to prefer the large outcome in any condition (see Tables 6 and 7 for full statistics). (c) Shown are flavour-selectivity indices with the same conventions as inb, with insets showing the indices in the trials immediately after flavour shifts. Indices were not shifted towards either flavour in any condition, but like controls had a larger magnitude (absolute value) and were more likely to be significant, in the preferred direction compared with the anti-preferred, late in blocks. In the preferred direction, flavour indices were significantly larger in magnitude in the lesion group compared with the sham group consistent with a stronger representation of flavour after OFC lesions. choc., chocolate; van., vanilla. 1a and Supplementary Table 4 for the same analyses using t-statistics). The development of the bias is consistent with it being an effect of training. Notably, index scores comparing firing on the basis of reward flavour showed a similar pattern, with flavour selectivity in the neurons’ preferred directions developing with training after a flavour switch. This pattern was not evident in the average population response because both flavours were equally represented across the population ( Fig. 3c ). However, to the extent that flavour-selectivity was present, its magnitude (as measured by the absolute value of the flavour index) was greater in the preferred direction than in the anti-preferred direction, late in blocks. See Table 3 for full statistics on flavour-selectivity indices. Table 2 Number selectivity in cue-selective neurons recorded in sham rats, statistics. Full size table Table 3 Flavour selectivity in cue-selective neurons recorded in sham rats, statistics. Full size table Thus, overall, cue-evoked activity in VS of sham rats was highly associative. We replicated earlier findings showing that this activity was strongly driven by the required response direction and the number of the predicted outcome. Further, we found that while flavour information was integrated into this single-unit value/direction representation, there was relatively little encoding of the predicted outcome flavour independent of its number. Indeed, only 3 of 66 neurons exhibited a main effect of flavour in their firing without any additional effect of number ( Fig. 2c ), a fraction of units that is not significantly different from chance (by chi-square test, P =0.74). OFC lesions eliminate reward-number representations The pattern of activity observed in cue-responsive units was dramatically altered when OFC was lesioned unilaterally on the side of the recording electrode. Although the prevalence (26/193 units) of cue-responsive neurons in VS was unaffected by the lesions, these units were much more likely to respond to specific flavours independent of their number ( Fig. 2f,h ). Across the population, there was less number selectivity independent of flavour, and much more flavour selectivity independent of number ( Fig. 2d ). Indeed, only one neuron exhibited a pure number-related response (with no additional effect of flavour), a proportion that is not significantly different from chance (by chi-square test, P =0.90). See Table 1 for a full accounting of neuron categorization and statistics. The effects of OFC lesions were also evident in the population response, which while showing a robust cue response, was not biased to fire to the large reward as a population, in either the preferred or anti-preferred direction ( Fig. 4 ; see Table 4 for full statistics; see Supplementary Fig. 2a for the same analyses using t-statistics). Number indices comparing firing on the basis of reward number confirmed this lack of representation; late in blocks in the preferred direction, the mean index score (using either the subtraction index or a t-statistic) was not significantly shifted away from zero, and the number of significantly selective neurons (four small-preferring versus four large-preferring) was equally distributed. In addition, a direct comparison of the t-statistic showed that number-selectivity indices of the populations in lesion and sham rats were significantly different (see Supplementary Table 6 for full statistics). 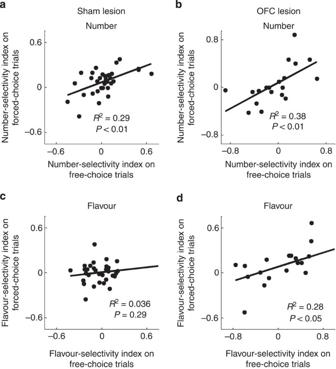Figure 6: Number-selectivity indices measured on free-choice trials were correlated with those on forced-choice trials, in both the sham and OFC-lesion groups. Flavour-selectivity indices were uncorrelated in the sham group but correlated in the OFC-lesion group. Scatter plots show (a,b) number-selectivity indices on free-choice and matched forced-choice trials in each neuron’s preferred side or (c,d) the corresponding flavour-selectivity indices. Neurons were only included when recorded in sessions with at least one free-choice trial in each condition on the preferred side. The effect of lesions on number encoding could also be seen by comparing the development of number-selectivity with changes in choice behaviour after number switches: in shams, average number indices showed a steady increase paralleling the development of choice rate towards the newly large side; in the lesion group, average number indices were unstable at the beginning of blocks and failed to show a steady increase ( Fig. 5 ; see Supplementary Fig. 3 for the same analyses using t-statistics). Figure 4: Outcome selectivity in ventral striatum of OFC-lesioned rats. ( a ) Shown are population averages of normalized firing rate across the time of the trial, aligned to the end of the odour period, for all odour-responsive units ( n =26). Activity is averaged by preferred (left panel) and anti-preferred (right panel) directions, and by the specific reward available at the end of the trial (in different colours). Preferred direction was defined for each unit by the direction with the highest average activity during the epoch from odour initiation to response initiation (in grey shading). Only correct forced-choice trials in the latter part of the block (after the first 20 correct trials) are included in the averages. There were no bins with significant (sig.) effects of number or flavour (flav), by ANOVA on a sliding average of five bins across neurons. ( b ) Shown are number-selectivity indices during the odour epoch for each neuron in the population, separately for the preferred (left panels) and anti-preferred (right panels) directions. Insets show indices early in blocks immediately following number shifts. Number-selectivity index was defined as the difference in normalized firing rate between conditions with the large reward and those with the small reward. Dark-coded units are those in which this difference was significant across trials. Unlike in controls, indices were not more likely to prefer the large outcome in any condition (see Tables 6 and 7 for full statistics). ( c ) Shown are flavour-selectivity indices with the same conventions as in b , with insets showing the indices in the trials immediately after flavour shifts. Indices were not shifted towards either flavour in any condition, but like controls had a larger magnitude (absolute value) and were more likely to be significant, in the preferred direction compared with the anti-preferred, late in blocks. In the preferred direction, flavour indices were significantly larger in magnitude in the lesion group compared with the sham group consistent with a stronger representation of flavour after OFC lesions. choc., chocolate; van., vanilla. 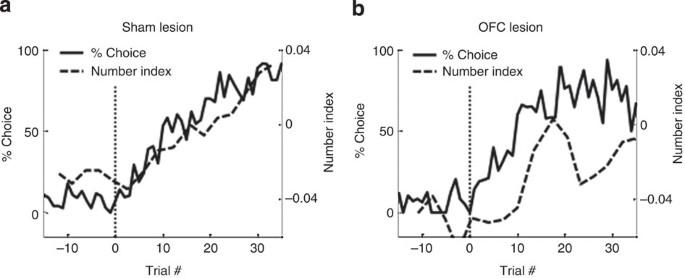Full size image Table 4 Number selectivity in cue-selective neurons recorded in lesion versus sham rats, statistics. Figure 5: Number-selectivity of VS cue-responsive neurons develops with choice performance after number switches in the sham group but not in the OFC-lesion group. The solid lines show the average percentage of choice of the side on which the large reward was delivered after the block switch (marked by the vertical dotted line). Only free-choice trials that occurred at each trial position of the block were included. The dashed lines show the average number-selectivity index for the comparison of a sliding group of 10 forced-choice trials towards the side on which the large reward was delivered around a number block switch minus the corresponding 10 forced-choice trials towards the same side when the small reward was delivered. Each index value was aligned with the average trial number, relative to the block switch, of the groups of trials with which it was calculated. (a) Shows this comparison for the control group and (b) for the OFC lesion group. All cue-responsive neurons were included. Full size table Figure 5: Number-selectivity of VS cue-responsive neurons develops with choice performance after number switches in the sham group but not in the OFC-lesion group. The solid lines show the average percentage of choice of the side on which the large reward was delivered after the block switch (marked by the vertical dotted line). Only free-choice trials that occurred at each trial position of the block were included. The dashed lines show the average number-selectivity index for the comparison of a sliding group of 10 forced-choice trials towards the side on which the large reward was delivered around a number block switch minus the corresponding 10 forced-choice trials towards the same side when the small reward was delivered. Each index value was aligned with the average trial number, relative to the block switch, of the groups of trials with which it was calculated. ( a ) Shows this comparison for the control group and ( b ) for the OFC lesion group. All cue-responsive neurons were included. Full size image In lesioned rats, flavour encoding was similar to that in shams, in that, (1) it was equally distributed between chocolate-preferring and vanilla-preferring, (2) it developed across the block and (3) it was of greater magnitude (that is, absolute value of the flavour indices) and more likely to be significant in the preferred direction compared with the anti-preferred. However, it was different than that in shams in that there was a greater proportion of flavour-selective neurons (as mentioned earlier), and the magnitude of indices was greater in the lesioned rats. Thus, ipsilateral OFC lesions not only altered and reduced number-related activity, it also seemed to increase flavour-related activity in VS neurons. See Supplementary Table 7 for full statistics on flavour-selectivity indices, and see Supplementary Fig. 2b and Supplementary Table 8 for the corresponding analyses using t -statistics. Activity on free-choice trials Free-choice trials were included primarily as a way to monitor behaviour. It is difficult to analyse the influence of reward and direction on neural activity on these trials, because after learning there is a large asymmetry in the number of choices towards the large versus small reward ( ∼ 85% large choice). Nevertheless, it is worth asking whether the firing patterns observed on forced-choice trials described above are similar on free-choice trials. To address this question, we identified 33 and 19 cue-responsive neurons in sham and lesioned rats, respectively, that were recorded in sessions in which the rat made at least one free-choice response after learning in the neuron’s preferred direction in each block. When data from each neuron’s preferred direction were considered, the outcome-index scores of these neurons on free-choice trials were significantly correlated with the scores on forced-choice trials, with the exception of flavour-selectivity indices in shams ( Fig. 6 ). These results suggest that the firing patterns observed on forced-choice trials are generally also present in the less reliable free-choice data. Figure 6: Number-selectivity indices measured on free-choice trials were correlated with those on forced-choice trials, in both the sham and OFC-lesion groups. Flavour-selectivity indices were uncorrelated in the sham group but correlated in the OFC-lesion group. Scatter plots show ( a , b ) number-selectivity indices on free-choice and matched forced-choice trials in each neuron’s preferred side or ( c , d ) the corresponding flavour-selectivity indices. Neurons were only included when recorded in sessions with at least one free-choice trial in each condition on the preferred side. Full size image Here, we recorded single-unit activity in the VS core in rats performing an odour-guided choice task in which cues predicted different numbers of rewards—a feature related to value—or different flavours of rewards—a feature related to identity—across blocks of trials. Neurons recorded in sham-lesioned rats exhibited differential activity to the cues that reflected information about the expected reward. This activity integrated information about the response required and the value of the expected reward, either alone or in combination with its identity, with relatively little representation of identity alone. Neurotoxic lesions of the OFC ipsilateral to the recording electrode did not affect the proportion of cue-evoked firing nor did it diminish its directional or cue-selectivity; however, the cue-selectivity was more heavily influenced by reward identity and much less by value. These results demonstrate that the OFC plays a strong role in shaping cue-evoked activity in the VS core. Input from OFC seems to bias what are otherwise largely neutral associative representations reflecting sensory information to represent this information in conjunction with its value or biological significance. Thus, in shams, there was significant coding of reward number independent of flavour and an over-representation of the cues predictive of the larger, more valuable reward. Without input from ipsilateral OFC, these representations became more neutral. This was evident in an increase in the number of neurons that responded simply on the basis of the flavour or identity of the predicted reward; however, it was also evident in the loss of the bias in signalling the larger reward. Notably, the loss of this bias was not due to a loss in signalling on the basis of reward number; the prevalence of number-selective neurons was not different between the two groups when those with a flavour interaction were included in the count, and the absolute value of number-selectivity index scores (either subtraction or t-statistic) across the population was also not different between the groups. Instead, the number selectivity was simply no longer biased towards the larger reward in the lesion group. In other words, number became more like the other features (flavour, response direction) that continued to be signalled by VS core neurons in the lesioned rats. What are the implications of this finding? First, it is important to note that, while the OFC projects directly to this region of VS, it also influences processing in a host of other regions, such as amygdala and ventral tegmental area, through which OFC output could impact processing in VS indirectly. Thus, the effects of the lesions may be due to the loss of either direct or indirect influence of output from the OFC on processing in VS. Indeed given how strongly these areas are linked, it is particularly interesting that much of the cue-evoked activity in VS was not dependent on the OFC. Overall phasic firing to the cues was largely unaffected, as was the proportion that showed differential activity; it was only the information content of that firing that was shifted. Second, it is important to note that we used lesions to remove the influence of OFC. Lesions allow for downstream compensation, thus it is possible that over time the VS reorganized to become more sensory specific and less general in the process. This seems somewhat unlikely given that some of the above studies used lesions to disrupt the behaviours, but it cannot be ruled out. The lesions were also unilateral, thus there was preserved processing in the contralateral hemisphere. It is possible that part of the compensation might have even involved strengthening of crossed connections, thus it is possible that the effects of bilateral lesions would be qualitatively different. These caveats aside, the current results are novel given the apparent differential involvement of VS core and OFC in behaviours such as PIT and unblocking, in which behaviour can be driven by either the general value of Pavlovian cues or their ability to predict specific properties of the associated rewards [16] , [18] , [32] , [33] , [34] , [35] . OFC is clearly necessary for the latter process [32] , [33] , [34] , [35] , whereas the VS core is most commonly proposed to be involved only in the former [16] , [18] (but see ref. 34 ). On the basis of this apparent dichotomy, we expected OFC input to be important for maintaining the specificity of the representations, whereas our results appear to show the opposite. While the OFC has been implicated in specific PIT [33] , its role in general PIT has not been directly tested to the best of our knowledge. The current results suggest that it might be important for both. Further, the current results suggest that disconnection of lateral OFC and VS core might also impact general PIT. In addition, the current results provide novel insight into how input from OFC impacts processing in downstream areas. The impact of OFC input is subtle. Associative representations in VS core were not silenced by the irreversible loss of OFC input. Indeed, they remained largely unchanged in many ways. This is consistent with the relatively subtle effects of OFC damage on behaviour. Many, if not most, simple associative behaviours are not affected by OFC damage [36] . These results also highlight the importance of OFC to determining the biological significance of associative information. Although our design does not explicitly dissociate incidental and biologically meaningful associative information, the associations between the cues and the specific sensory properties of the outcomes would consist of both. The VS receives input from other areas, such as hippocampus, which might be able to signal associative information independent of its significance or value, and neurons in VS core have recently been shown to signal incidental associative information [37] . By contrast, the OFC would be more critical for driving the over-representation of specific sensory associations that have biological significance. This is consistent with lesion studies that have typically found that behaviours requiring predictions about the value of outcomes are affected by OFC lesions. That the loss of this information did not impact behaviour may reflect the over-training these rats had and/or the operation of the intact hemisphere. Notably, bilateral lesions of VS core have been shown to disrupt value-based changes in the speed of choice behaviour in this setting [38] . The current results suggest that these effects may reflect the loss of this shaping function of OFC input. Subjects Male Long–Evans rats were obtained at 175–200 g from Charles River Labs, Wilmington, MA. Rats were tested at the University of Maryland School of Medicine in accordance with SOM and NIH guidelines. Surgical procedures and histology Surgical procedures followed guidelines for aseptic technique. Electrodes, consisting of drivable bundles of eight 25-μm diameter FeNiCr wires (Stablohm 675, California Fine Wire, Grover Beach, CA) electroplated with platinum to an impedance of ∼ 300 kOhms, were manufactured and implanted as in prior recording experiments. Driveable electrodes were implanted bilaterally in VS (1.6 mm anterior to bregma, ±1.5 mm laterally, and, to begin, 6.0 mm ventral to the surface of the brain) in each rat. Neurotoxic or sham lesions were made by infusing NMDA (or just lowering a pipette) at four different positions in one hemisphere (at 4.0 mm anterior to bregma, 3.7 and 2.2 mm laterally, and at 3.0 mm anterior to bregma, 4.2 and 3.2 mm laterally; infusions consisted of 0.1 μl of 12.5 mg ml −1 NMDA solution in saline, except for the final position, which consisted of 0.05 μl of the same solution). Lesions were made in the left hemisphere in two rats, and the right hemisphere in the other three. Results of the neural analysis did not differ by location of lesion, and hence the two lesion groups were combined. Recorded units from hemispheres contralateral to lesions showed some characteristics in common with those from ipsilateral hemispheres; however, because the number of units from the contralateral side was relatively low ( n =139), we could not draw strong conclusions about the effects of contralateral versus ipsilateral lesions. Therefore, only units from the ipsilateral side were included in the final analysis. In sham rats, results did not differ by recorded hemisphere and hence both were included. At the end of the study, final electrode positions were marked, the rats were euthanized with an overdose of isoflurane and perfused and the brains were removed from the skulls and processed using standard techniques. Some sections from one sham and one lesioned rat were lost during a laboratory move; results did not differ in these rats versus other subjects nor did the main findings depend on their inclusion. Behavioural task Recording was conducted in aluminium chambers, on one wall of which was a panel with an odour port and two fluid wells arranged below it (see Fig. 1 ). The odour port was connected to an air flow dilution olfactometer to allow the rapid delivery of olfactory cues. The fluid wells were connected to fluid delivery lines containing flavoured milk (Nesquick brand chocolate or vanilla) diluted 50% with water. Delivery of odours at the odour port and the fluids at the fluid wells was controlled by a custom C++ programme interfaced with solenoid valves. Photobeam breaks at the port and wells were monitored and recorded by the programme. A houselight was also controlled by the programme. Rats were shaped to nose poke and respond at the fluid wells according to instructional odour cues before undergoing surgery to create lesions and implant electrodes. After recovery, we retrained rats to work with the recording cable. Each training session included as many trials as a rat would perform before quitting, ∼ 150–250. Recording was begun when rats could complete five blocks of trials (at least 260 trials) with the cable. Each recording session consisted of a series of self-paced trials organized into five blocks. Rats could initiate a trial by poking into the odour port while the houselight was illuminated. Beginning 500 ms after the odour poke, an odour would be delivered for 500 ms. If the rat withdrew from the odour port before completion of the 1,000 ms pre-odour+odour period, the trial would be aborted and the houselight turned off. At the end of the odour, rats could respond by moving from the odour port to the left fluid well or the right fluid well, after which they had to wait for 500 ms before fluid delivery began; if they exited the well during this period, no fluid was delivered and the trial ended. The identity of the odour specified whether they could receive reward at the left well (forced-choice left), the right well (forced-choice right) or either well (free-choice). The identity and meaning of these odours remained the same across the entire experiment. Odours were presented in a pseudorandom sequence such that the free-choice odour was presented on 7/20 trials and the left/right odours were presented in equal numbers (±1 over 250 trials). In addition, the same odour could be presented on no more than three consecutive trials. Rewards were either one bolus or three boli of chocolate or vanilla milk, with bolus number ∼ 0.05 ml and 500 ms between boli. Response-reward contingencies were consistent within blocks of trials, such that the same reward would be delivered for every correct right response, either free or forced choice, and a different reward would be delivered for every correct left response, free or forced choice. The reward schedule was arranged so that in each block, reward features available on one side were always paired with the opposite reward features on the other side—thus, when one drop of chocolate milk was available on the left, three drops of vanilla were available on the right and so on., resulting in a total of four different reward combinations. On the first block, which was used to set the rats’ expectations before the initial block switch, one of these combinations was randomly chosen. The subsequent four block transitions then followed in order: (1) a drop-number transition, in which the side with one drop changed to three drops and vice versa, but the side-flavour contingencies remained the same; (2) a flavour transition, in which the side with chocolate changed to vanilla and vice versa, but the side-number contingencies remained the same, (3) another drop-number transition, (4) another flavour transition. These block transitions were not explicitly signalled. During testing, rats were limited to 10 min of ad lib water each day, in addition to fluid earned in the task. Flavour preference testing In six rats from a separate experiment (same strain and source, and same water restriction regimen), we compared consumption of the chocolate versus vanilla milk solution in two-bottle tests. All the rats were tested for 10 total minutes, with the location of the bottles swapped every 30 s. Two rats were given five 2-min tests while the other four rats were given one 10-min test each. Single-unit recording Procedures were the same as described previously [39] . Wires were screened for activity daily; if no activity was detected, the rat was removed and the electrode assembly was advanced 40 or 80 μm. Otherwise, a session was conducted and the electrode was advanced by at least 40 μm at the end of the session. Neural activity was recorded using Plexon Multichannel Acquisition Processor systems (Dallas, TX), interfaced with odour discrimination training chambers. Signals from the electrode wires were amplified and filtered by standard procedures described in previous studies. Waveforms (>2.5:1 signal-to-noise) were extracted from active channels and recorded with event timestamps sent by the behavioural programme. Waveforms were not inverted before data analysis. Data analysis Units were sorted using Offline Sorter software from Plexon Inc. (Dallas, TX), using a template-matching algorithm. Sorted files were then processed in Neuroexplorer to extract unit timestamps and relevant event markers. These data were subsequently analysed in Matlab (Natick, MA). To analyse cue-evoked activity, we examined firing rate in the epoch between initiation of odour delivery and odour port exit. We first screened for odour-responsive neurons by testing, across all correct forced-choice trials, for units that showed a significant increase over baseline (defined as firing rate between 2 s before odour poke to 1 s before odour poke; t -test, P <0.05). Among these units, we next tested for effects of predicted outcome. We divided trials by whether they occurred before (early) or after (late) the twentieth correct trial in each block. We then assigned each unit’s preferred direction as that which had the highest average firing rate during the odour epoch on correct forced-choice trials occurring late in blocks. We performed an ANOVA with factors number (three drops or one drop) and flavour (chocolate or vanilla) on firing rate in the preferred direction, and for comparison, in the anti-preferred direction. Neurons were coded as significantly number encoding when there was an effect of number or an interaction of number with flavour, and significantly flavour encoding when there was an effect of flavour or an interaction of flavour with number ( α =0.05). An ANOVA with direction as an additional factor resulted in qualitatively similar results. To measure the degree of number- and flavour-selectivity, we calculated a number and flavour index for each neuron in each direction. To do so, we peak-normalized each neuron by dividing all the firing rates by a normalization factor, which was the peak firing rate across the trial in 500-ms bins after averaging across the first 10 and last 10 of each of the eight number-flavour-well conditions in the last four blocks. We then calculated the number and flavour indices separately in the preferred and anti-preferred directions as: Number index=average peak-normalized firing rate on all three-drop trials−average peak-normalized firing rate on all one-drop trials. Flavour index=average peak-normalized firing rate on all chocolate trials−average peak-normalized firing rate on all vanilla trials. For the ‘early’ condition, the above formulae only included trials occurring before the first 20 correct trials in blocks immediately after number switches for the number index and immediately after flavour switches for the flavour index. The ‘late’ condition included trials occurring after the first 20 in any block. We also recalculated all indices as the t-statistic resulting from the comparison of the two conditions across trials (for example, three-drop trials occurring after the first 20 in any block versus one-drop trials occurring after the first 20 in any block). We tested the development of number-selectivity at the start of blocks by calculating a moving average of the subtraction index and the t-statistic across all cue-responsive neurons, using a block of 10 trials in each condition before the block switch, and then stepping the blocks of 10 up by one trial, across the block. These moving averages were aligned to the average trial, relative to the block switch, across the trials that were used for each index or t-statistic and plotted against the choice percentage towards the large reward at the same trial position in the block. In the neural analyses described above forced-choice trials were used, because these trials were equally distributed between the two sides across all blocks. To examine encoding on free-choice trials, we matched free-choice trials with forced-choice trials occurring in the same block and direction, and approximately the same position within the block. Specifically, for each free-choice trial, we took the closest forced-choice trial that occurred before the free-choice trial (in the same direction and block) and the closest forced-choice trial that occurred after the free-choice trial (in the same direction and block) and averaged the binned firing rates between those two trials. We then compared indices based on free-choice trials with the corresponding indices based on the matched set of forced-choice trials. To test whether the population neural results were consistent across recordings from different rats, we performed separate ANOVAs with ‘rat’ as an additional factor (with neuron being the subject), and examined interactions between factors of interest and ‘rat’. Statistics were done using Matlab, Excel and Statistica. For displays of neural activity, bin-number was 100 ms. Neural activity in the displays was smoothed with a boxcar algorithm, with a three-bin boxcar for population plots and a nine-bin boxcar for single-unit plots. To display bin-by-bin effects of number or flavour, we calculated a sliding average of five bins and performed an ANOVA, separately for data from each side (across trials for the single-unit data, and across neurons for the population data). To meet significance, a set of bins had to be a part of at least three consecutive sliding bin-sets that showed a main effect (at P <0.05). Significant bin-sets were then plotted across the middle three bins for each set on the activity plots, separately for number and flavour main effects. To make plots of trial-by-trial choice rate ( Fig. 1 ), we first aligned all rewarded trials for all blocks, and for each trial (first, second, third and so on after the block switch) we took the proportion of choices towards the side with the three-drop reward, excluding all blocks in which a forced-choice trial happened to occur on that trial. The line was then smoothed using a three-bin boxcar, separately for before and after the switch. How to cite this article: Cooch, N. K. et al. Orbitofrontal lesions eliminate signalling of biological significance in cue-responsive ventral striatal neurons. Nat. Commun. 6:7195 doi: 10.1038/ncomms8195 (2015).